An electrochemical system for efficiently harvesting low-grade heat energy Efficient and low-cost thermal energy-harvesting systems are needed to utilize the tremendous low-grade heat sources. Although thermoelectric devices are attractive, its efficiency is limited by the relatively low figure-of-merit and low-temperature differential. An alternative approach is to explore thermodynamic cycles. Thermogalvanic effect, the dependence of electrode potential on temperature, can construct such cycles. In one cycle, an electrochemical cell is charged at a temperature and then discharged at a different temperature with higher cell voltage, thereby converting heat to electricity. Here we report an electrochemical system using a copper hexacyanoferrate cathode and a Cu/Cu 2+ anode to convert heat into electricity. The electrode materials have low polarization, high charge capacity, moderate temperature coefficients and low specific heat. These features lead to a high heat-to-electricity energy conversion efficiency of 5.7% when cycled between 10 and 60 °C, opening a promising way to utilize low-grade heat. Low-grade heat sources (<100 °C) are ubiquitous, generated in energy conversion and utilization processes [1] , [2] . Among the methods for converting this energy to electricity, thermoelectric (TE) materials and devices have been studied extensively for several decades [3] , [4] , [5] , [6] , [7] , [8] , [9] . Despite recent progress, however, the figure of merit (ZT) of thermoelectrics is limited to 2 at high temperatures and 1.5 below 100 °C [10] , [11] . Seebeck effect in electrochemical system is also investigated for thermal energy harvesting in similar architectures as a TE device, but the efficiency achieved is usually lower than 0.5% below 100 °C since the thermopower is limited by poor ionic conductivity of electrolyte, which is more than three orders of magnitude smaller than the electronic conductivity in state-of-the-art TE materials [12] , [13] , [14] , [15] . An alternative approach of electrochemical system for thermal energy harvesting is to explore thermodynamic cycle as in thermomechanical engines. Here we report an efficient thermally regenerative electrochemical cycle (TREC) based on the thermogalvanic effect, temperature dependence of electrode potential. For a half-cell reaction, A+n e − →B, the temperature coefficient is defined as where V is the electrode potential, T is temperature, n is the number of electrons transferred in the reaction, F is Faraday’s constant and Δ S A,B is the partial molar entropy change for the half-cell reaction in isothermal condition (see Supplementary Note 1 ). This effect indicates that the voltage of a battery depends on temperature; thus a thermodynamic cycle can be constructed by discharging the battery at T 1 and charging back at T 2 . If the charging voltage at T 2 is lower than the discharging voltage at T 1 , net energy is produced by the voltage difference, originating from heat absorbed at the higher temperature, similar to a thermomechanical engine with the Carnot efficiency as the upper limit. In practice, instead of transport property limited in TE devices, the efficiency of TREC is limited by the heat capacity of materials and effectiveness of heat exchangers [16] . The concept of TREC was developed a few decades ago for high-temperature applications (500–1,500 °C) and showed efficiency of 40–50% of the Carnot limit. But, low-temperature TREC did not received as much attention since electrode materials with low polarization and high charge capacity at low temperature were limited [17] . Hammond and William [18] tested an aqueous redox couple for low-temperature solar-thermal applications, but the precipitation of reactants, large internal resistance and poor solubility of active redox species causing large heat capacity of the system prevented them from reporting device operational characteristics and measuring the device efficiency, although a high efficiency was theoretically projected based on the measured open-circuit voltage OCV and 100% heat recuperation assumption. The recent development of highly reversible electrode materials with very low polarization loss during the research of rechargeable batteries has now made it possible for us to exploit the TREC concept in a new way. Here we present a high-efficiency TREC for harvesting low-grade heat energy by employing solid copper hexacyanoferrate (CuHCF) as a positive electrode and Cu/Cu 2+ as a negative electrode in an aqueous electrolyte. The fast kinetics, high charge capacity, high-temperature coefficient (α) and low heat capacity of these materials allow the system to operate with excellent efficiency. Working principle of TREC To harvest thermal energy, the entire device undergoes a thermal cycle containing four processes: heating up, charging, cooling down and discharging ( Fig. 1a ). This cycle is also plotted on a temperature–entropy (T–S) diagram to clarify the thermodynamics ( Fig. 1b ). In process 1, the cell is in the discharged state and heated from T L to T H (low to high temperature) at open circuit. Since CuHCF has a negative α and Cu/Cu 2+ has a positive α , the OCV of the full cell decreases during this process. The cell is then charged at a low voltage at T H in process 2, and the entropy of the cell increases through heat absorption during the electrochemical reaction. In process 3, the cell is disconnected and cooled from T H to T L , and thus the OCV increases. In the final process, the cell is discharged at a higher voltage at T L , and the entropy of the cell decreases through the ejection of heat into the environment. After the cycle, the system returns to the original discharged state at T L . Since the charging voltage is lower than the discharging voltage, net work ( W ) is extracted as the difference between charging and discharging energy. This is the opposite of the consumption of energy due to electrochemical hysteresis during a typical charge/discharge cycle of a battery, since the charging energy here is partially provided by heat ( Supplementary Fig. 1 ). Such a conversion process of thermal energy into electrochemical energy requires that the electrochemical voltage hysteresis during charge/discharge at a fixed temperature is much smaller than the voltage difference caused by temperature change, calling for the highly reversible electrochemical electrodes. 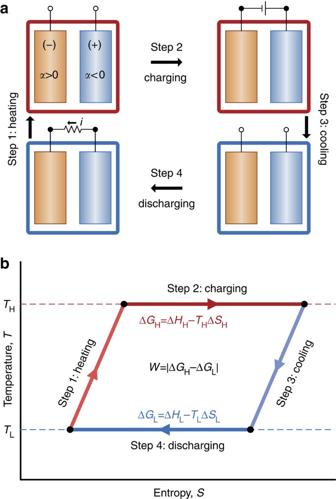Figure 1: Working principle of TREC for thermal energy harvesting. (a) Schematic view of thermal cycling: process 1, heating up the cell; process 2, charging at high temperature; process 3, cooling down the cell; process 4, discharging at low temperature. (b) Temperature–entropy (T–S) diagram of thermal cycling assuming a temperature range betweenTLandTH. The theoretical energy gained over one cycle is the area of the loop determined by the temperature difference and entropy change. Figure 1: Working principle of TREC for thermal energy harvesting. ( a ) Schematic view of thermal cycling: process 1, heating up the cell; process 2, charging at high temperature; process 3, cooling down the cell; process 4, discharging at low temperature. ( b ) Temperature–entropy (T–S) diagram of thermal cycling assuming a temperature range between T L and T H . The theoretical energy gained over one cycle is the area of the loop determined by the temperature difference and entropy change. Full size image The efficiency of the system ( η ) is calculated as the net work ( W ) divided by the thermal energy input. If the enthalpy change Δ H and the entropy change Δ S are the same at T H and T L , which is a good approximation when Δ T =( T H − T L ) is small, the maximum W is Δ T Δ S ( Fig. 1b ). The energy input to complete the cycle includes two parts: the heat absorbed at T H ( Q H = T H Δ S ) and the external heat required to raise the temperature of the system ( Q HX ). As part of heat rejected from the cooling process can be used for the heating process through heat recuperation, Q HX can be expressed as Q HX =(1− η HX ) C p Δ T , where C p is the total heat capacity of the electrochemical cell and η HX is the efficiency of the heat recuperation (See Supplementary Fig. 2 and Supplementary Note 2 ). Consequently η can be expressed as: where E loss is the energy loss due to the cell electrical resistance. Note that Δ T Δ S = αQ c Δ T , where Q c is the charge capacity of the battery and α is the temperature coefficient of the electrochemical cell. The efficiency can be written as where I is the current used in discharging and charging. R H and R L are the internal resistance at T H and T L , respectively. Y = αQ c / C p , is a dimensionless parameter to describe the requirements of the system for high efficiency. A thorough derivation of efficiency is presented in Supplementary Notes 3 and 4 . If only the contributions of the electrode materials are considered, and it is assumed that both electrodes have the same properties except opposite signs of the temperature coefficient, Y = αq c / c p and it is defined as the figure of merit of an electrode material for TREC, but not thermocells. Here, q c is the specific charge capacity and c p is the specific heat of an electrode. Consequently, it is clear that a higher temperature coefficient ( α ), a higher specific charge capacity ( q c ) and a smaller specific heat ( c p ) lead to higher efficiency for heat-to-electricity conversion. In addition, low-voltage polarization and effective heat recuperation can also improve the efficiency. The value of Y for individual materials can be negative or positive, depending on the sign of the temperature coefficient, although efficiency expression takes its absolute value. Electrochemical system for harvesting thermal energy Considering these requirements, we have selected solid CuHCF as the positive electrode for the TREC because of its negative temperature coefficient (−0.36 mV K −1 ), high specific charge capacity (60 mAh g −1 ) compared with redox couples in solution, relatively low specific heat (1.07 JK −1 g −1 ), and ultra-low voltage hysteresis [19] , [20] , [21] . The corresponding figure of merit Y is as high as −0.073. For the negative electrode, a copper metal immersed in 3 M Cu(NO 3 ) 2 aqueous solution is selected because of the high positive temperature coefficient (0.83 mV K −1 ) of Cu/Cu 2+ and its large specific charge capacity (825 mAh g −1 Cu). Although the corresponding Y for Cu alone is as high as 6.55, the electrolyte is an active component in the full cell and its contribution to heat capacity is considerable. Including the electrolytes, the corresponding Y are −0.031 and 0.125 for CuHCF/6 M NaNO 3 and Cu/3 M Cu 2+ , respectively. Y for the full cell reaches −0.068 with both electrolyte and electrode considered (see Supplementary Table 1 and Supplementary Note 5 ). The relevant redox reactions at each electrode are Na 0.71 Cu[Fe III (CN) 6 ] 0.72 + a(Na + +e − )=Na 0.71+a Cu[Fe III (CN) 6 ] 0.72−a [Fe II (CN) 6 ] 0.72+a and Cu 2+ +2e − =Cu. The temperature coefficient of each electrode was tested by measuring the OCV while varying temperature from 10 to 70 °C. 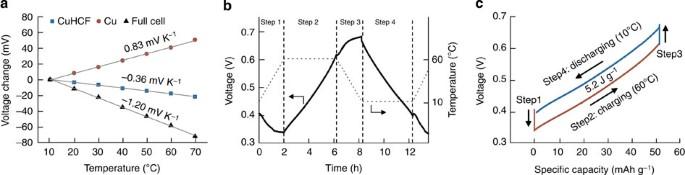Figure 2: The electrochemical system for harvesting thermal energy with CuHCF and Cu/Cu2+electrodes. (a) Voltage change of the CuHCF electrode, the Cu electrode and the full cell compared with the initial voltage at 10 °C when the temperature varies from 10 to 70 °C. The slopes of the fitting lines (grey) represent the temperature coefficients of electrodes and the full cell. (b) Voltage plot of the cell during one cycle of thermal energy harvesting when the temperature is varied between 10 and 60 °C and the current density is 7.2 mA g−1. The temperature of each process is shown by the grey-dotted line, which is artificially superimposed for clarity. (c) A voltage plot of the cell versus the specific charge capacity of CuHCF during one cycle with the same conditions as inb. The red line represents heating (process 1) and charging (process 2) of the cell at 60 °C, and the blue line represents cooling (process 3) and discharging (process 4) of the cell at 10 °C. Figure 2a shows the OCV change of the CuHCF electrode (50% state of charge), the Cu/Cu 2+ (3 M) electrode and the full cell for each 10-°C increment when the voltage is set at 0 V at 10 °C. The potentials of both electrodes exhibit a linear dependence on temperature, indicating a constant α in the temperature window tested. The measured temperature coefficients of CuHCF, Cu/Cu 2+ and the full cell are −0.36, 0.83 and −1.20 mV K −1 , respectively. These experimental values match with the expected ones. Figure 2b shows the voltage versus time plot of the full cell over one thermal cycle between 10 and 60 °C when the specific current density is 7.2 mA g −1 with respect to active materials (All current, energy and power densities are based on the mass of active materials, including CuHCF, electrolyte for Na + , copper and water for Cu 2+ in this paper.). In process 1, the OVC of the cell decreases from 0.406 to 0.337 V as the temperature increases from 10 to 60 °C. Then the cell is charged for 250 min at 60 °C in process 2 and the voltage gradually increases. In process 3, the OCV of the cell increases from 0.613 to 0.679 V as the temperature decreases back to 10 °C. The cell is discharged in process 4 at 10 °C until the voltage reaches the initial voltage of the discharged state at the beginning of process 1. The corresponding plot of voltage against specific charge capacity based on the mass of CuHCF is shown in Fig. 2c . The average charging voltage is 59.0 mV lower than the average-discharging voltage and thus electrical energy is generated with a net energy density of 5.2 J g −1 . The voltage spikes at the beginning of each process are electrochemical in nature and are due to overpotential and internal resistance. At the end of process 4, the discharging curve forms nearly perfect closed loop with only tiny loss of electric charges. The Coulombic efficiency (ratio of the amount of charge extracted during discharging to that of adding in during charging) for this cycle is adequately high ~\n98.6%. Figure 2: The electrochemical system for harvesting thermal energy with CuHCF and Cu/Cu 2+ electrodes. ( a ) Voltage change of the CuHCF electrode, the Cu electrode and the full cell compared with the initial voltage at 10 °C when the temperature varies from 10 to 70 °C. The slopes of the fitting lines (grey) represent the temperature coefficients of electrodes and the full cell. ( b ) Voltage plot of the cell during one cycle of thermal energy harvesting when the temperature is varied between 10 and 60 °C and the current density is 7.2 mA g −1 . The temperature of each process is shown by the grey-dotted line, which is artificially superimposed for clarity. ( c ) A voltage plot of the cell versus the specific charge capacity of CuHCF during one cycle with the same conditions as in b . The red line represents heating (process 1) and charging (process 2) of the cell at 60 °C, and the blue line represents cooling (process 3) and discharging (process 4) of the cell at 10 °C. Full size image Efficiency of TREC The efficiency of the cycle is estimated based on equation (2). Effects of internal resistance and Coulombic efficiency are both taken into account. Details of calculations are shown in Supplementary Note 4 and Supplementary Fig. 3 . 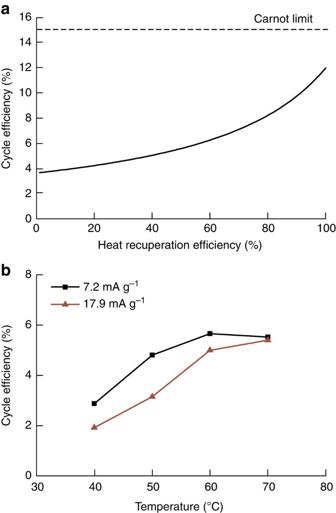Figure 3: Efficiency of TREC. (a) Efficiency of the cell cycle versus heat recuperation efficiency to be potentially included in the system when the temperature range is between 10 and 60 °C and the current density is 7.2 mA g−1. Grey-dotted line represents the theoretical Carnot efficiency. (b) Efficiency of the cell for various high temperatures (TH) from 40 to 70 °C and two current densities, 7.2 and 17.9 mA g−1, when the low temperature (TL) is fixed at 10 °C and 50% heat recuperation efficiency is included in the calculation. Figure 3a plots the cycle efficiency versus the efficiency of heat recuperation when cycled between 10 and 60 °C. The current density is 7.2 mA g −1 . When heat recuperation is not used, the cycle efficiency is 3.7%. The final system efficiency could be much higher when heat recuperation is used, depending on the efficiency of the heat recuperation system ( η HX ). We have designed and tested two heat recuperation schemes using dummy cells and commercial battery cells, since the current laboratory cell is too small to match the heat exchanger size. The test combined with thermal modelling shows that heat recuperation efficiency ( η HX ) between 45–80% can be achieved (details are shown in Supplementary Note 6 ). In the following, we will assume 50% heat recuperation efficiency to discuss the cycle efficiency, which we believe is a conservative number. With 50% heat recuperation efficiency, the corresponding cycle efficiency increases to 5.7%. Figure 3b shows the efficiency at various cycling conditions with T H varying between 40 and 70 °C and T L fixed at 10 °C. At a current density of 7.2 mA g −1 and η HX =50%, the cycle efficiencies are 2.9% for T H =40 °C, 4.8% for 50 °C, 5.7% for 60 °C and 5.5% for 70 °C. The efficiency becomes higher as T H increases because of larger voltage difference between the charging and discharging curves and faster kinetics at higher temperature. However, this tendency changes between a T H of 60 and 70 °C, since the Coulombic efficiency of CuHCF starts to decrease at these temperatures. When the temperature is higher than 80 °C, significant decrease of Coulombic efficiency leads to rapid drop of the cycle efficiency (see Supplementary Fig. 4 ). When the current density increases to 17.9 mA g −1 for higher power output, the cycle efficiencies are still as high as 1.9% for T H =40 °C, 3.2% for 50 °C, 5.0% for 60 °C and 5.4% for 70 °C despite the larger overpotential. The efficiency is much higher than previous reports on thermogalvanic cells ( Supplementary Table 2 ). Figure 3: Efficiency of TREC. ( a ) Efficiency of the cell cycle versus heat recuperation efficiency to be potentially included in the system when the temperature range is between 10 and 60 °C and the current density is 7.2 mA g −1 . Grey-dotted line represents the theoretical Carnot efficiency. ( b ) Efficiency of the cell for various high temperatures ( T H ) from 40 to 70 °C and two current densities, 7.2 and 17.9 mA g −1 , when the low temperature ( T L ) is fixed at 10 °C and 50% heat recuperation efficiency is included in the calculation. Full size image Long-term cycling The cycling performance of the thermal energy-harvesting system is shown in Fig. 4a . T H and T L are set to 50 °C and 20 °C to represent widely accessible temperatures of waste heat and room temperature, respectively. The current density is 17.9 mA g −1 . The energy density reaches 1.26 J g −1 in the initial cycle with an efficiency of 1.8%. The average efficiency is 1.7% ( η HX =50%). 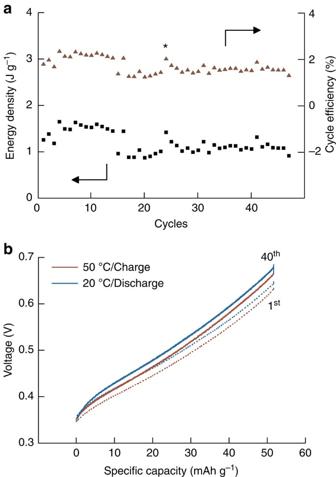Figure 4: Cycling performance of the thermally regenerative electrochemical system with CuHCF and Cu/Cu2+electrodes. (a) Measured energy density and corresponding efficiency when 50% heat recuperation efficiency is included in the calculations. The cell is cycled between 20 and 50 °C and the current density is 17.9 mA g−1. The asterisk denotes changing of the electrolyte because of drying after the 24th cycle. (b) Voltage plot of the cell versus specific charge capacity of CuHCF during the 1st (dotted line) and 40th (solid line) cycles under the same conditions as ina. The red and blue lines represent charging at 50 °C and discharging at 20 °C, respectively. Figure 4b compares the full-cell voltage versus specific capacity of CuHCF for the 1st and 40th cycle. A slight shift of the loop is observed, but there is no significant change in the overall shape. In addition, the cycling performance of CuHCF at higher temperature is confirmed by long-term galvanostatic cycling of a CuHCF electrode at 70 °C. At this temperature, the capacity decay is only 9.1% over 500 cycles ( Supplementary Fig. 5 ). This result signifies that this TREC for thermal energy harvesting is expected to have stable cycling with further optimization. Figure 4: Cycling performance of the thermally regenerative electrochemical system with CuHCF and Cu/Cu 2+ electrodes. ( a ) Measured energy density and corresponding efficiency when 50% heat recuperation efficiency is included in the calculations. The cell is cycled between 20 and 50 °C and the current density is 17.9 mA g −1 . The asterisk denotes changing of the electrolyte because of drying after the 24th cycle. ( b ) Voltage plot of the cell versus specific charge capacity of CuHCF during the 1st (dotted line) and 40th (solid line) cycles under the same conditions as in a . The red and blue lines represent charging at 50 °C and discharging at 20 °C, respectively. Full size image Since TE devices are major candidates for waste heat recovery, it is useful to point out the differences between TE devices and TREC. The ZT of TE materials are determined by transport properties, while the thermogalvanic figure of merit Y is determined by thermodynamic properties. TE devices can have high-power density, provided that one can manage heat flow on both hot and the cold sides to create the needed temperature difference, while TREC has relatively low-power density. Its power density depends on applied current density and voltage gap between charging and discharging of a cycle. We have estimated a power density of 1.2 mW g −1 for cell operating between 10–80 °C at current density of 58.5 mA g −1 with a 1-hour cycling time, based on the mass of all active materials and electrolytes (see Supplementary Fig. 6 ). Further improvement in power density can be realized by optimizing device configuration, utilizing porous copper electrode, and exploring new system with fast kinetics and large temperature coefficient (see Supplementary Note 7 ). On the other hand, due to its constant temperature operation, thermal management challenges, which are crucial for low-grade waste heat utilization, can be easier, as we have demonstrated in the heat recuperation testing ( Supplementary Figs 7–13 and Supplementary Table 3 ). With such an understanding first, we can now convert the efficiency achieved in TREC into familiar ZT in TE materials. The estimated ZT is 3.5 for the efficiency of 5.7% when temperature is varied from 10 to 60 °C, current density is 7.2 mA g −1 and η HX =50% is considered in the calculation. When the current density increases to 17.9 mA g −1 (close to current density for maximum power density), the efficiency is 5.0% and the estimated ZT is 2.7. In this study, a thermally regenerative electrochemical system with CuHCF and Cu/Cu 2+ electrodes is developed for low-grade thermal energy harvesting. The electrode materials have large temperature coefficients, high charge capacity, low specific heat and small hysteresis. These properties lead to a high thermogalvanic figure of merit (Y) for the electrode materials and thus excellent heat-to-electricity conversion efficiency: a cycle efficiency of 3.7% between 10 and 60 °C without any heat recuperation and 5.7% when 50% heat recuperation is assumed. The achieved cycle efficiency still has room to improve by improving heat recuperation efficiency and reducing the amount of electrolyte through increasing the concentration of salts [22] , [23] . Furthermore, the efficiency improvement in this system is possible by searching for materials with higher figure of merit and smaller hysteresis, especially solid electrode materials with a positive temperature coefficient as a counter electrode to CuHCF. In addition, further optimization is needed to improve the power output while maintaining high efficiency of thermal energy harvesting. Our work points to the great potential of TREC for utilizing ubiquitous low-temperature heat sources. Material synthesis and electrode preparation CuHCF was synthesized by a simple co-precipitation method. In total, 40 mM of Cu(NO 3 ) 2 and 20 mM of K 3 Fe(CN) 6 (Sigma Aldrich) were prepared in 120 ml of distilled water, then both solutions were simultaneously added in drops into 60 ml of deionized-water under vigorous stirring. A yellowish green precipitate formed during the precipitation. Then, the solid precipitate was filtered and washed several times with deionized-water. Afterward, the precipitate was dried in vacuum oven at 40 °C for 12 h. The diameter of as-formed particles is typically below 100 nm ( Supplementary Fig. 14 ) To prepare electrodes, a mixture of 70% wt/wt CuHCF, 20% wt/wt amorphous carbon (Timcal Super P Li) and 10% wt/wt polyvinylidene fluoride (Kynar HSV 900) was grounded by hand. 1-methyl-2-pyrrolidinone was added in the mixture to form slurry, which was spread on carbon cloth current collector (Fuel Cell Earth). The mass loading of CuCHF was between 2 and 3 mg on area of about 0.25 cm 2 . Electrochemical characterizations TREC is demonstrated as form of a flooded beaker cell as shown in Supplementary Fig. 3B . CuHCF on carbon cloth (~\n0.25 cm 2 ) is connected to working electrode. Cu foil (~\n4 cm 2 ) is connected to counter electrode. In total, 6 M NaNO 3 and 3 M Cu(NO 3 ) 2 electrolytes are used for CuHCF and Cu electrodes, respectively. These electrolytes are separated by three anion exchange membranes (Selemion DSV, AGC engineering, LTD, Japan). Ag/AgCl in saturated KCl solution is located between the membranes as a reference electrode. Electrochemical test of the cell is performed by a potentiostat with 50 μV resolution (VM3, BioLogic). During the measurement, recording voltage was fluctuating ±0.2 mV due to noise. The temperature measurement uncertainty is estimated to be ±0.2 °C as we wait until equilibrium in an environment chamber (BTU-133, ESPEC North America, INC.), while the precision of the thermometer is ±0.1 °C.’ The overall relative uncertainty in efficiency is estimated to be less than 3%, which corresponds to less than 0.2% in the absolute conversion efficiency. Specific heat measurement The specific heat ( c p ) of the CuHCF was measured by differential scanning calorimetry test after drying the sample at 40~\n50 °C for more than 24 h. The measurements were carried out by differential scanning calorimetry Q100 (TA instrument). The measurement range was 20–70 °C with the ramping rate of 5 °C min −1 . The heat flow curve is shown in Supplementary Fig. 15 . The calculated c p of CuHCF is 1.07 J g −1 K −1 . Efficiency calculation The thermal-to-electricity efficiency is based on experimental charge/discharge curves of TREC cells. The specific heat is calculated based on experimental measurements. More details can be found in Supplementary Notes 3 and 4 . How to cite this article: Lee, S. W. et al. An electrochemical system for efficiently harvesting low-grade heat energy. Nat. Commun. 5:3942 doi: 10.1038/ncomms4942 (2014).